Cascade cyclization of alkene-tethered acylsilanes and allylic sulfones enabled by unproductive energy transfer photocatalysis Developing photo-induced cascade cyclization of alkene-tethered acylsilanes is challenging, because acylsilanes are unstable under light irradiation. Herein, we report that the energy transfer from excited acylsilanes to a photocatalyst that possesses lower triplet energy can inhibit the undesired decomposition of acylsilanes. With neutral Eosin Y as the photocatalyst, an efficient synthesis of cyclopentanol derivatives is achieved with alkene-tethered acylsilanes and allylic sulfones. The reaction shows broad substrate scope and the synthetic potential of this transformation is highlighted by the construction of cyclopentanol derivatives which contain fused-ring or bridged-ring. Organosilicon compounds are important molecules in chemistry and material science, due to their less toxic and easy-to-handle properties and the abundance of silicon element [1] , [2] , [3] , [4] . As a kind of unique carbonyl compounds, acylsilanes have been widely used in synthetic chemistry [5] , [6] , [7] , [8] , [9] . Compared to common ketones, acylsilanes can absorb relatively longer wavelength light, and they usually possess lower triplet energies than ketones (e.g. 3-phenyl-1-(trimethylsilyl)propan-1-one, E T = 55.3 kcal/mol; benzophenone, E T = 69.1 kcal/mol) [10] , [11] . Although the early studies pioneered by Brook and co-workers focused on the photochemical studies of acylsilanes with UV light [12] , [13] , [14] , recent work found that they are labile under visible-light irradiation, sometimes in the presence of a photocatalyst, resulting in the formation of carbenes A or acyl radicals B (Fig. 1a ) [10] , [15] , [16] , [17] , [18] , [19] , [20] , [21] , [22] , [23] , [24] , [25] . For example, Priebbenow disclosed a visible-light-induced intramolecular [2 + 1] cycloaddition of acylsilanes with tethered alkenes (Fig. 1b ) [23] . Recently, we developed the photocatalyzed intramolecular [2 + 1] cycloaddition of acylsilanes with olefins (Fig. 1c ) [24] . In this context, it is challenging to develop a photo-induced cascade cyclization reaction of alkene-tethered acylsilanes with another reaction partner [26] , [27] , [28] , because of the undesired decomposition of acylsilanes under light irradiation (Fig. 1a ). Glorius [10] , Kusama [18] and our group [24] , [25] have reported that carbene generation from acylsilanes could be facilitated through the energy transfer catalysis with photocatalysts which possess higher triplet energies than those of the corresponding acylsilanes [29] , [30] , [31] , [32] , [33] , [34] , [35] , [36] , [37] , [38] , [39] , [40] , [41] , [42] , [43] , [44] . Inspired by these works, we envisioned that the inhibition of light-induced decomposition of acylsilanes might be achieved via energy transfer from the excited acylsilanes to a photocatalyst that possesses lower triplet energy (Fig. 1d ). Under the guidance of this concept, we have developed an efficient photocatalyzed synthesis of cyclopentanol derivatives with alkene-tethered acylsilanes and allylic sulfones (Fig. 1d ). Fig. 1: Background and our strategy for the synthesis of cyclopentanols enabled by inhibition of light-induced decomposition of acylsilanes through energy transfer catalysis. a Previous work: acylsilanes are unstable under light irradiation. b Priebbenow’s intramolecular [2 + 1] cyclization of acylsilanes with tethered olefins. c Our intermolecular [2 + 1] cyclization of acylsilanes with olefins. d This work: visible-light-induced cascade cyclization of acylsilanes and allylic sulfones. Full size image It is worth noting that cyclopentanol is an important structural motif in bioactive molecules. The commercially available drugs such as Levonorgestrel, Faslodex and Remodulin all contain cyclopentanol motif and the sales of these three drugs all exceeded 500 million dollars in 2020 [45] . Therefore, the development of novel synthetic methodologies for the construction of cyclopentanol motif is of great value. In recent years, photocatalyzed radical cyclization has emerged as powerful strategy to construct cyclic compounds, and toxic reagents are often not necessary under these conditions [46] , [47] , [48] , [49] , [50] , [51] . However, previous synthesis of cyclopentanols through intramolecular radical cyclization to acylsilanes relied on thermal chemistry [52] , [53] , [54] . In this work, we successfully employed acylsilanes in photocatalyzed multicomponent radical cyclization reaction to synthesize complex cyclopentanols. The reaction shows broad substrate scope and the synthetic potential of this transformation is highlighted by the synthesis of fused-ring and bridged-ring compounds. The success of the reaction is attributed to the energy transfer from excited acylsilanes to the photocatalyst that possesses lower triplet energy which inhibits the undesired decomposition of acylsilanes. This work will pave the way to develop new ground state reactions of acyl silanes under photochemical conditions. Evaluation of reaction conditions We commenced our study by testing our proposal about the inhibition of light-induced decomposition of acylsilanes via energy transfer catalysis. Firstly, we tested the conversion of acylsilane 1a in CDCl 3 (Fig. 2a ). It was found that 1a gradually decomposed under white light. However, the addition of 1 mol% of neutral Eosin Y dramatically decreased the conversion of 1a . The control experiment confirmed that 1a is stable in dark conditions and no conversion was observed in the absence of light after 30 h. The results of luminescence quenching experiments confirmed that the excited state of 1a could be quenched with different concentrations of Eosin Y (Fig. 2b ). We can see from the UV-vis spectrum that there is no significant overlap between 1a and Eosin Y absorbance (Fig. 2c ). Moreover, transient absorption measurements have been conducted to investigate the possible triplet-triplet energy transfer from 1a to Eosin Y. We found that the sample which contain both 1a and Eosin Y showed strong T 1 → T n transition of Eosin Y at around 580 nm, which was much stronger than the signal in the sample with only Eosin Y. These results strongly support the involvement of triplet-triplet energy transfer process between 1a and Eosin Y, which is consistent to the lower triplet energy of neutral Eosin Y ( E T = 43.6 kcal/mol) [55] than that of acylsilane 1a ( E T = 56.7 kcal/mol) (For the details on the calculation of the triplet energy of acylsilane 1a , see the Supporting Information.). Encouraged by the above results, we then applied the concept of inhibition of light-induced decomposition of acylsilanes via energy transfer from excited acylsilanes to neutral Eosin Y in the synthesis of cyclopentanol derivatives. 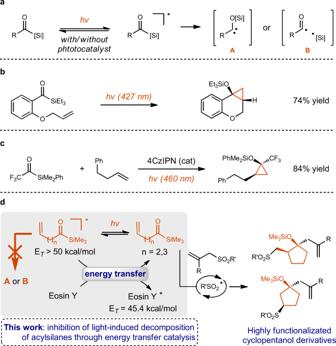Fig. 1: Background and our strategy for the synthesis of cyclopentanols enabled by inhibition of light-induced decomposition of acylsilanes through energy transfer catalysis. aPrevious work: acylsilanes are unstable under light irradiation.bPriebbenow’s intramolecular [2 + 1] cyclization of acylsilanes with tethered olefins.cOur intermolecular [2 + 1] cyclization of acylsilanes with olefins.dThis work: visible-light-induced cascade cyclization of acylsilanes and allylic sulfones. The investigation of reaction conditions was performed with alkene-tethered acylsilane 1a and allylic sulfone 2a as the model substrates under photocatalysis conditions (Table 1 ). We found that when neutral Eosin Y (1 mol%) was used as the catalyst in the presence of KOPiv (1 equiv.) as base, the reaction between acylsilane 1a (2 equiv. ), allylic sulfone 2a (1 equiv.) and PhSO 2 Na (0.2 equiv.) in MeCN/H 2 O (v/v = 1/3, 0.067 M) at room temperature under white LEDs (6 W) for 12 h generated product 3a in 89% yield with 90/10 dr (isolated in 82% yield, Table 1 , entry 1). Cyclohexanol derivative 4a , acylation product 5a and [2 + 1] cyclization product 6a were not detected. Without neutral Eosin Y, there was only 14% yield of 3a , while 91% conversion of 1a was observed, indicating the importance of the neutral Eosin Y in the protection of 1a from undesired decomposition (Table 1 , entry 2). The use of Ru(bpy) 2 Cl 2 ( E T = 46.5 kcal/mol, E 1/2 (*Ru II /Ru I ) = 0.77 V in MeCN vs SCE) [29] as the photocatalyst resulted in decreased yield of 3a and conversion of 1a , probably because of its low oxidation potential and the lower triplet energy than acylsilane 1a , (Table 1 , entry 3). The use of fac -Ir(ppy) 3 ( E T = 57.8 kcal/mol) [29] , 4CzIPN ( E T = 59.6 kcal/mol) [56] or FIrPic ( E T = 60.5 kcal/mol) [26] as the photocatalyst resulted in decreased yield of 3a , probably because their relatively higher triplet energies than that of 1a would promote the decomposition of 1a to carbene intermediate (Table 1 , entries 4 ∼ 6). Meanwhile, the formation of acylation product 5a could be explained by the oxidation-induced C-Si bond homolysis to generate acyl radical, due to the higher oxidation ability of excited 4CzIPN and FIrPic (4CzIPN, E 1/2 (PC*/PC˙ˉ) = 1.43 V in MeCN vs SCE; [57] FIrPic, E 1/2 (*Ir III /Ir II ) = 1.40 V in MeCN vs SCE [26] ; neutral Eosin Y, E 1/2 ( 3 EY*/EY - ) = 0.83 V in MeCN vs SCE [58] ; 1a , E 1/2 = 1.23 V in MeCN vs SCE [For the details on the cyclic voltammograms of the acylsilanes used in this study, please see the Supporting Information]). The above proposal was further supported by the experimental result with 9-mesityl-10-methylacridinium perchlorate ( E T = 44.7 kcal/mol [59] ; E 1/2 (PC*/PC˙ˉ) = 2.06 V in MeCN vs SCE [60] ) as the catalyst, in which, significantly decreased conversion of 1a and increased yield of 5a were obtained (Table 1 , entry 7). Control experiments revealed that the use of MeCN/H 2 O mixture was important for the high yield of the reaction (Table 1 , entries 8 and 9). Without light, there was less than 2% conversion of acylsilane 1a (Table 1 , entry 10). PhSO 2 Na and KOPiv were not necessary for the success of the reaction, but the addition of them indeed increased the efficiency, which might because they can promote the generation of PhSO 2 radical (Table 1 , entries 11 and 12). Further study confirmed that the reaction is sensitive to air, supporting that the reaction might proceed through a radical mechanism (Table 1 , entry 13). Fig. 2: Proof of concept: inhibition of visible-light-induced decomposition of acylsilanes via energy transfer catalysis. a Light-induced decomposition of 1a . b Luminescence quenching experiments. c UV/Vis of 1a and Eosin Y. d Transient absorption spectra observed after laser excitation (λ ex = 355 nm) of system containing (green line) 1 mM 1a (black line), 0.1 mM Eosin Y and (red line) 1 mM 1a + 0.1 mM Eosin Y. Source data are provided as a Source Data file. Full size image Table 1 Investigation of reaction conditions a Full size table Scope of the reaction With the optimal reaction conditions in hand, we investigated the reaction scope for the synthesis of β -substituted cyclopentanol derivatives with acylsilane 1a as the reagent (Fig. 3 ). Firstly, we tested the influence of silyl groups on the efficiency of the reaction. The small SiMe 3 was found to be better than SiEt 3 , SiMe 2 ( t -Bu), SiMe 2 Ph and SiMePh 2 , although all of them afforded the desired product in more than 50% yield, and the diastereoselectivity was not significantly affected. A variety of allylic sulfones could be employed as the substrates, affording compounds 3 f ~ 3aa in 52%~95% yield, with up to 99/1 dr. The Csp 2 -Me, Csp 2 -F, Csp 2 -Cl, Csp 2 -Br, Csp 2 -I, Csp 2 -OMe, Csp 2 -CF 3 , Csp 3 -CN bonds were tolerated, affording products 3 f ~ 3o and 3t in 55~95% yield. In addition, cyclopropane-containing compound 3p was synthesized in 88% yield with 99/1dr. Electron-rich thienyl and furyl groups were tolerated ( 3q , 82% yield, 90/10 dr; 3r , 85% yield, 89/11 dr). Moreover, primary alcohol ( 3w , 82% yield, 90/10 dr), tertiary alcohol ( 3x , 88% yield, 92/8 dr), aliphatic aldehyde ( 3 y , 80% yield, 90/10 dr) have been successfully synthesized, further highlighting the functional group tolerance of the reaction. Two examples of the synthesis of bioactive molecular derivatives have also been achieved, indicating the synthetic potential of the reaction ( 3z , 56% yield, 80/20 dr, 3aa , 52% yield, 93/7 dr). Fig. 3: Scope for the synthesis of β-substituted cyclopentanol derivatives. a Total yield of the isolated two diastereoisomers is reported. b neutral Eosin Y (2 mol%), KOPiv (1.5 equiv. ), 36 h. c 3a (0.05 mmol), TBAF (1 M in THF, 0.1 mmol), rt, 0.5 h. Full size image It is worthy to note that the cyclopentyl siloxanes could be easily converted to cyclopentanols through the desilylation with TBAF, and 3a’ was obtained in 97% yield with 90/10 dr with 3a as the starting material. The relative configuration of the major isomer of 3j was determined by X-Ray Crystal Structure Analysis [61] , and the configuration of other products were assigned accordingly. After achieving the efficient synthesis of β -substituted cyclopentanol derivatives with 1a as the reagent, we applied the cascade cyclization reaction in the synthesis of γ -substituted cyclopentyl siloxanes with acylsilane 1 f (Fig. 4 ). Various five-membered ring products were synthesized in moderate yields, although the diastereoselectivities were generally low ( 7a ~ 7i , 48%~71% yield, 50/50~65/35 dr). Again, the reaction tolerated Csp 2 -Me, Csp 2 -F, Csp 2 -Cl, Csp 2 -Br, Csp 2 -I, Csp 2 -OMe, Csp 2 -CF 3 bonds. Electron-rich furyl group-containing compound 7 g was isolated in 71% yield, and the naphthyl-group containing product 7 h was obtained in 51% yield. In all cases, we did not observe any four-membered ring product. When TBAF was used to quench the reaction, cyclopentanol 7a’ was isolated in 60% yield, 53/47 dr. Fig. 4: Scope for the synthesis of γ-substituted cyclopentanol derivatives. a Total yield of the isolated two diastereoisomers is reported. b Yield of the alcohol after desilylation with TBAF is reported. c neutral Eosin Y (2 mol%), KOPiv (1.5 equiv. ), 36 h. Full size image Since only catalytic amount of PhSO 2 Na was needed to facilitate the above reaction (Fig. 3 ), we wondered whether our reaction could be applied in the synthesis of different functionalized sulfones by modification of the allylic sulfones. We found that the reactions performed efficiently for the synthesis of β -substituted cyclopentyl siloxanes in the presence of only 2~5 mol% of PhSO 2 Na (Fig. 5 ). Compounds 3ab ~ 3ag were synthesized in 54~87% yield with 84/16~95/5 dr. However, 2 equivalents of ArSO 2 Na was needed to promote the reaction for the synthesis of γ -substituted cyclopentyl siloxanes, indicating their less efficiency in the completion of the catalytic cycles. Fig. 5: Scope for the synthesis of different sulfonyl group-substituted cyclopentanol derivatives. a Total yield of the isolated two diastereoisomers is reported. b ArSO 2 Na (20 mol%) was used. c PhSO 2 Na (5 mol%) was used. d ArSO 2 Na (2 equiv.) was used, MeOH/H 2 O = 1/2 (v/v). Full size image Synthetic transformations of compound 3a and 7a It is worthy to note that cyclopentanols containing fused-ring and bridged-ring motifs are widely found in bioactive molecules. For example, compound Y is a Na + K + -ATPase inhibitor and compound Z is an adenosine receptor antagonist [62] , [63] . Taking the advantage of the strong electron-withdrawing group ability of the sulfonyl group, the deprotonation-conjugate addition reaction of compound 3a has been achieved, affording fused-ring compound 8 in 82% yield with >99:1 dr. With compound 7a as the substrate, bridged-ring compound 9 was synthesized in 74% yield with >99:1 dr (Fig. 6 ). The facile construction of these two types of compounds with the cyclization products demonstrated the synthetic potential of the current methodology. Fig. 6: Down-stream transformations. Fused ring compound 8 and bridged ring compound 9 were successfully prepared with cyclization products 3a and 7a , respectively. Full size image Mechanistic study Preliminary studies have been conducted to understand the possible mechanism (Fig. 7 ). The addition of 1 equivalent of TEMPO completely inhibited the reaction of 1a and 2a , and compound X was detected by HRMS, indicating that PhSO 2 radical might participated in the catalytic cycle (Fig. 7a ). The time profile of the light on/off experiments over time supported that the reaction might proceed through radical chain reaction (Fig. 7b ). In addition, the reaction could proceed in dark after light irradiation for 10 min (Fig. 7b ). The quantum yield around 1.5 also supported the radical chain mechanism (Fig. 7b ). The Stern-Volmer fluorescence-quenching experiments validated the interaction of neutral Eosin Y with both allylic sulfone 2a and PhSO 2 Na, which were two possible pathways to generate PhSO 2 radical (Fig. 7c ). However, we cannot rule out the possibility of generation of PhSO 2 radical through the sensitization of 2a with excited acylsilane or direct homolysis of 2a under light irradiation. In addition, PhSO 2 Na can be oxidized by excited neutral Eosin Y to generate PhSO 2 radical [64] . The importance of ArSO 2 Na in the reaction for the synthesis of γ -substituted cyclopentanol derivatives indicated that ArSO 2 radical was more likely generated from ArSO 2 anion first. When E -stilbene ( E T = 51.0 kcal/mol) [65] was added to the reaction, only 24% yield of cascade cyclization product was obtained and the isomerization of E -stilbene to Z -stilbene was observed, supporting the energy transfer from excited acylsilane to E -stilbene (Fig. 7d ). Fig. 7: Mechanism study. a Reaction in the presence of TEMPO indicates that PhSO 2 radical might participated in the reaction. b Light on-off experiments, determination of quantum yield and light-darkness control experiment support that the reaction might proceed through radical chain mechanism. c Eosin Y emission quenching by 2a and Eosin Y emission quenching by PhSO 2 Na. The Stern-Volmer fluorescence-quenching experiments validate the interaction of neutral Eosin Y with both allylic sulfone 2a and PhSO 2 Na. d Reaction in the presence of E -stilbene instead of Eosin Y supports the energy transfer from excited acylsilane to E -stilbene. Source data are provided as a Source Data file. Full size image Density functional theory (DFT) calculations were then carried out to study the radical chain mechanism and the selectivity control in the cascade cyclization of alkene-tethered acylsilane 1a with allylic sulfone 2a . As shown in Fig. 8 , the radical addition of PhSO 2 radical to the terminal carbon of alkene (via TS-1a ) generates a secondary carbon-centered radical 10a . The activation free energy is 3.2 kcal/mol lower than the formation of primary carbon-centered radical 10b (via TS-1b ). Radical cyclization (via TS-2a or TS-2b ) is demonstrated to be the regioselectivity-determining step. The irreversible formation of five-membered ring through TS-2a is kinetically favored due to the higher stability of the secondary carbon-centered radical. From oxygen-centered radical 11a , the radical Brook rearrangement occurs easily through TS-3a (Δ G ‡ = 3.8 kcal/mol), leading to the formation of a stable tertiary carbon-centered radical. Subsequent Giese-type radical addition towards electron-deficient alkene 2a controls the diastereoselectivity. The steric clash evidenced by the H•••H distance of 2.23 Å in TS-4b renders the formation of radical 13b kinetically disfavored (ΔΔ G ‡ = 4.7 kcal/mol), resulting in the selective formation of trans product. Finally, the β -scission of alkyl radical 13a generates the five-membered cyclization product 3a and regenerates the PhSO 2 radical. Fig. 8: Computational study of the radical chain mechanism in PhSO 2 radical involved cascade cyclization of alkene-tethered acylsilane 1a and allylic sulfone 2a. All energies were calculated at M06-2X/6-311 + G(d,p)/SMD(water)//M06-2X/6-31 G(d) level of theory. Full size image Based on these experimental and computational results, a possible mechanism was proposed in Fig. 9 . The energy transfer from the excited acylsilane to neutral Eosin Y inhibited the undesired decomposition of acylsilane 1a under the photocatalysis conditions and keep enough acylsilane in ground state to participate in the reaction with PhSO 2 radical. The generation of more stable secondary carbon radical 10a is favorable over primary carbon radical 10b . The intramolecular addition of 10a to the acylsilane would generate alkoxyl radical 11 , followed by radical Brook rearrangement to generate 12 [66] , [67] , [68] , [69] , [70] , [71] , [72] , [73] , [74] , [75] , [76] . Giese-type addition of 12 to allylic sulfone would generate intermediate 13 , which would eliminate PhSO 2 radical and product 3a to close mechanism cycle. Mechanistic studies revealed that the formation of five-membered cyclization product is promoted by the higher stability of secondary carbon-centered radical and the formation of trans product is promoted by the steric repulsion in Giese addition. As for the reactions with 1 f , 2 equivalents of ArSO 2 Na was needed to get high yield, indicating that radical chain process was less efficient than the reaction with 1a (for the DFT calculations and the proposed mechanism, see supporting information). Fig. 9: Proposed mechanism. 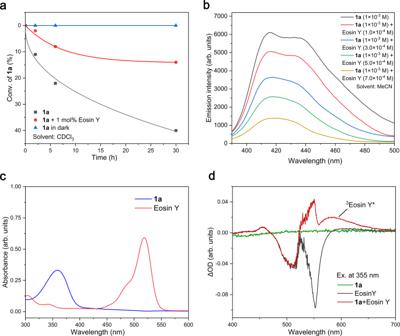Fig. 2: Proof of concept: inhibition of visible-light-induced decomposition of acylsilanes via energy transfer catalysis. aLight-induced decomposition of1a.bLuminescence quenching experiments.cUV/Vis of1aand Eosin Y.dTransient absorption spectra observed after laser excitation (λex= 355 nm) of system containing (green line) 1 mM1a(black line), 0.1 mM Eosin Y and (red line) 1 mM1a+ 0.1 mM Eosin Y. Source data are provided as a Source Data file. The unproductive energy transfer from excited acylsilane to Eosin Y inhibited the light-induced decomposition of acylsilanes, enabling the desired cascade cyclization reaction to generate cyclopentanol derivatives. Full size image In summary, we have developed a visible-light-induced cascade cyclization reaction of alkene-tethered acylsilanes with allylic sulfones. The reaction shows broad substrate scope, enabling the synthesis of various β-substituted and γ-substituted cyclopentanol derivatives. The synthetic potential of the transformation is highlighted by the construction of fuse-ring and bridge-ring compounds. The success of the reaction is attributed to the inhibition of undesired decomposition of acylsilanes through energy transfer from excited acylsilanes to the photocatalyst which possesses lower triplet energy. Previously, energy transfer has been mainly used in facilitating excitation state chemistry of acylsilanes, the strategy disclosed here would contribute to the design of more ground state reaction of acylsilanes under photocatalysis conditions. Typical procedure 1 ( 3a ). In a glovebox, to an oven-dried 10 mL tube was added 2a (28.6 mg, 0.1 mmol), PhSO 2 Na (3.2 mg, 0.02 mmol, 0.2 equiv. ), Eosin Y (0.65 mg, 0.001 mmol, 1 mol%), KOPiv (14.2 mg, 0.1 mmol, 1 equiv. ), MeCN/H 2 O = 1:3 (0.067 M) and 1a (34.0 mg, 0.2 mmol, 2 equiv.) sequentially. The tube was sealed, then irradiated with 6 W white LED lamps. The mixture was stirred under white light irradiation at ambient temperature for the 12 h. Then the light was turned off. The resulting mixture was filtered through a thin silica gel plug with EA (30 mL) as the eluent. 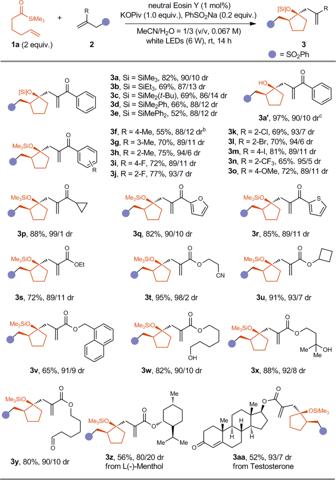Fig. 3: Scope for the synthesis of β-substituted cyclopentanol derivatives. aTotal yield of the isolated two diastereoisomers is reported.bneutral Eosin Y (2 mol%), KOPiv (1.5 equiv.), 36 h.c3a (0.05 mmol), TBAF (1 M in THF, 0.1 mmol), rt, 0.5 h. The organic phase was concentrated under reduced pressure. 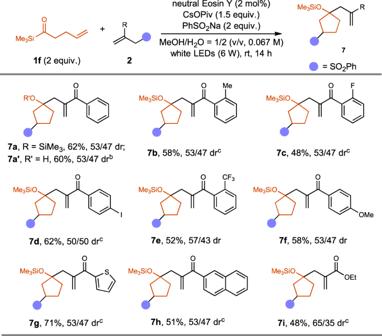Fig. 4: Scope for the synthesis of γ-substituted cyclopentanol derivatives. aTotal yield of the isolated two diastereoisomers is reported.bYield of the alcohol after desilylation with TBAF is reported.cneutral Eosin Y (2 mol%), KOPiv (1.5 equiv.), 36 h. The dr was determined by the analysis of the unpurified crude mixture by 1 H NMR. The crude product was purified with column chromatography on silica gel (300 ∼ 400 mesh) with PE/EA = 5/1 (v/v) as eluent to afford the title compound as a colorless oil (37.5 mg, 82% yield in total, a mixture of two disteraosiomers). 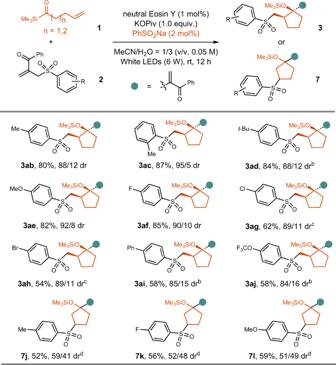Fig. 5: Scope for the synthesis of different sulfonyl group-substituted cyclopentanol derivatives. aTotal yield of the isolated two diastereoisomers is reported.bArSO2Na (20 mol%) was used.cPhSO2Na (5 mol%) was used.dArSO2Na (2 equiv.) was used, MeOH/H2O = 1/2 (v/v). Typical procedure 2 (7a) . In a glovebox, to an oven-dried 10 mL tube was added 2a (28.6 mg, 0.1 mmol), PhSO 2 Na (32.8 mg, 0.2 mmol, 2 equiv. ), Eosin Y (1.3 mg, 0.002 mmol, 2 mol%), CsOPiv (35.1 mg, 0.15 mmol, 1.5 equiv. 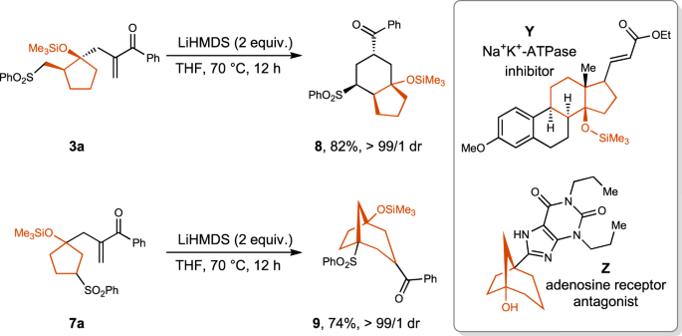Fig. 6: Down-stream transformations. Fused ring compound8and bridged ring compound9were successfully prepared with cyclization products3aand7a, respectively. ), MeOH/H 2 O = 1:2 (0.067 M) and 1 f (31.2 mg, 0.2 mmol, 2 equiv.) sequentially. The tube was sealed, then irradiated with 6 W white LED lamps. The mixture was stirred under white light irradiation at ambient temperature for the 12 h. Then the light was turned off. The resulting mixture was filtered through a thin silica gel plug with EA (30 mL) as the eluent. The organic phase was concentrated under reduced pressure. 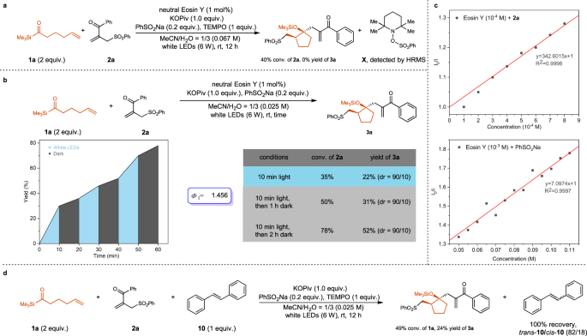Fig. 7: Mechanism study. aReaction in the presence of TEMPO indicates that PhSO2radical might participated in the reaction.bLight on-off experiments, determination of quantum yield and light-darkness control experiment support that the reaction might proceed through radical chain mechanism.cEosin Y emission quenching by2aand Eosin Y emission quenching by PhSO2Na. The Stern-Volmer fluorescence-quenching experiments validate the interaction of neutral Eosin Y with both allylic sulfone2aand PhSO2Na.dReaction in the presence ofE-stilbene instead of Eosin Y supports the energy transfer from excited acylsilane toE-stilbene. Source data are provided as a Source Data file. 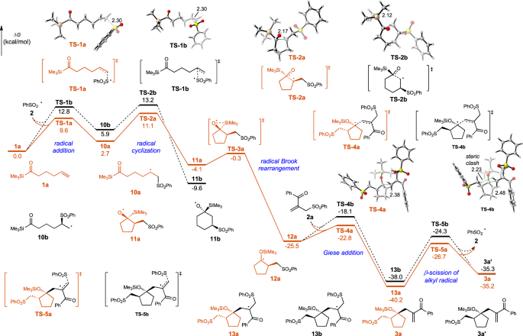Fig. 8: Computational study of the radical chain mechanism in PhSO2radical involved cascade cyclization of alkene-tethered acylsilane 1a and allylic sulfone 2a. All energies were calculated at M06-2X/6-311 + G(d,p)/SMD(water)//M06-2X/6-31 G(d) level of theory. 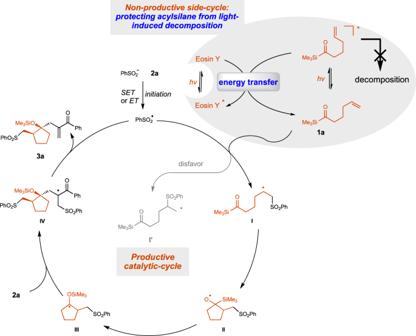Fig. 9: Proposed mechanism. The unproductive energy transfer from excited acylsilane to Eosin Y inhibited the light-induced decomposition of acylsilanes, enabling the desired cascade cyclization reaction to generate cyclopentanol derivatives. The crude product was purified with column chromatography on silica gel (300 ∼ 400 mesh) with PE/EA = 5/1 (v/v) as eluent to afford the title compound as a colorless oil (27.5 mg, 62 % yield in total, a mixture of two diastereoisomers).